Coordination tuning of cobalt phosphates towards efficient water oxidation catalyst The development of efficient and stable water oxidation catalysts is necessary for the realization of practically viable water-splitting systems. Although extensive studies have focused on the metal-oxide catalysts, the effect of metal coordination on the catalytic ability remains still elusive. Here we select four cobalt-based phosphate catalysts with various cobalt- and phosphate-group coordination as a platform to better understand the catalytic activity of cobalt-based materials. Although they exhibit various catalytic activities and stabilities during water oxidation, Na 2 CoP 2 O 7 with distorted cobalt tetrahedral geometry shows high activity comparable to that of amorphous cobalt phosphate under neutral conditions, along with high structural stability. First-principles calculations suggest that the surface reorganization by the pyrophosphate ligand induces a highly distorted tetrahedral geometry, where water molecules can favourably bind, resulting in a low overpotential ( ∼ 0.42 eV). Our findings emphasize the importance of local cobalt coordination in the catalysis and suggest the possible effect of polyanions on the water oxidation chemistry. Splitting water into hydrogen and oxygen molecules via solar energy has been considered as one of the most environment-friendly ways to effectively use renewable energy resources from harvest to redistribution [1] , [2] , [3] , [4] , [5] , [6] . Although it has been studied for more than a half century, the inefficiency of the oxygen evolution reaction (OER) has not yet been resolved and is still regarded as a bottleneck in the integration of an overall water splitting system [1] , [2] , [3] , [4] , [5] , [6] , [7] , [8] . This inefficiency is primarily due to the rigid O–O double bond formation and the sluggish proton-coupled electron-transfer reactions [7] , [8] , [9] . Noble-metal catalysts, such as Pt, IrO x and RuO x , exhibit outstanding OER catalytic activity; however, the high costs of these catalysts prohibit their practical use [10] , [11] , [12] , [13] , [14] . In this regard, the development of cost-effective, abundant-element-based and efficient OER catalysts is highly demanded. Inspired from the Mn-based water oxidation complex in photosystem II that generates oxygen from water with an exceptionally high efficiency [15] , [16] , [17] , numerous OER catalysts have been synthesized and evaluated using relatively cheaper 3 d transition metals (Mn, Fe, Co and Ni) [8] , [18] , [19] , [20] , [21] , [22] , [23] , [24] , [25] , [26] , [27] , [28] , [29] , [30] , [31] , [32] , [33] , [34] , [35] , [36] . In particular, cobalt-containing catalysts have been studied as promising OER catalysts because of their high catalytic activity for water oxidation, which is comparable to those of precious-metal-based catalysts [8] , [23] , [24] , [25] , [26] , [27] , [28] , [29] , [30] , [31] , [32] , [33] , [34] , [35] , [36] . Various cobalt-based oxides, perovskites and layered double hydroxides have been developed and examined via experimental and theoretical approaches [23] , [24] , [25] , [26] , [27] , [28] , [29] , [30] , [31] , [32] , [33] , [34] , [35] , [36] . Among these materials, cobalt phosphate (Co-Pi) prepared using electrodeposition exhibits one of the highest performances to date with efficient and stable catalytic performance [8] . The extraordinary performance of Co-Pi has cast fundamental questions on the correlation between cobalt chemistry and the OER mechanism, and has further promoted the exploration of other cobalt-based OER catalysts. Although various cobalt-based materials have been investigated as OER catalysts, researches were carried out mostly on materials with specific cobalt local environments such as octahedral ( O h ) cobalt [8] , [26] , [27] , [28] , [32] , [33] , [34] . Even amorphous Co-Pi has been recently shown to adopt the local O h coordination of cobalt [26] . Although the coordination and corresponding electronic structure of the transition metal in the catalysts is believed to greatly affect the OER activity [19] , [20] , [21] , [22] , [23] , [31] , [32] , [33] , [34] , there is a lack of systematic information relating the local cobalt coordination to the OER catalysis. Moreover, in practice, most of the cobalt-based materials reported thus far have been prone to transform into amorphous Co-Pi or cobalt-oxide-like phases from the surface under the typical pH and voltage regions where the OER proceeds [27] , [28] , [29] , [30] , [31] . This transformation makes it more difficult to apprehend the correlation between the structural cobalt geometry and the OER mechanisms, which has in turn retarded the development of new cobalt-based OER catalysts. Transition metal phosphates have positive attributes in structural stability, especially in oxidative environments over oxides, and can adopt versatile structures with various orientations of the phosphate group present in the crystal [37] , [38] , [39] . 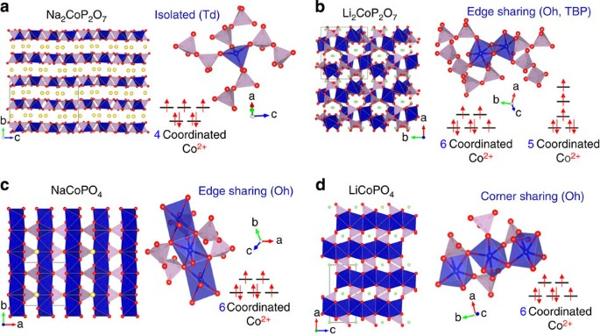Figure 1: Crystal structure and cobalt crystal field of cobalt phosphate catalysts. Crystal structures of (a) Na2CoP2O7, (b) Li2CoP2O7, (c) NaCoPO4and (d) LiCoPO4. The inset shows the local environment around the cobalt subunit (blue) and the spin state of the cobalt atom. The phosphate units, Na atoms and Li atoms are depicted in grey, yellow and green, respectively. As shown in Supplementary Table 1 , whereas conventional oxide materials have cobalt O h geometry with higher-symmetry crystal structures, phosphate/pyrophosphate-containing compounds have various cobalt geometries including tetrahedral ( T d ), trigonal bipyramidal (TBP) and O h , with lower-symmetry crystal structures due to the bulky phosphate/pyrophosphate ligands. Moreover, the flexible coordination of phosphate groups can stabilize the intermediate state of the transition metal by changing their local positions with ease, ensuring an effective redox change in the transition metal [20] , [40] . Indeed, our recent study using Mn 3 (PO 4 ) 2 ·3H 2 O as a OER catalyst demonstrated that the inherently unstable Mn(III) state is stabilized by the structural flexibility of the phosphate group [20] . Along with the case of Co-Pi [30] , it implies that the interplay between the transition metal and phosphate groups in the structure can also affect the catalytic activity, which, if clearly understood, would aid in the discovery of new efficient OER catalysts. Herein, we explore the OER catalytic capabilities of four cobalt-based phosphate materials with various cobalt environments, Na 2 CoP 2 O 7 , NaCoPO 4 , Li 2 CoP 2 O 7 and LiCoPO 4 , which are well known as cobalt redox-active electrode materials in rechargeable lithium or sodium batteries [41] , [42] , [43] , [44] , [45] . Except for LiCoPO 4 , other three materials have not been evaluated as OER catalysts. All of these materials have crystal structures in which cobalt polyhedrons are cross-linked by phosphate groups. The uniqueness of this selection of materials lies in the various local cobalt coordination, including O h , T d and TBP configurations, with different networks between the cobalt polyhedron. These different cobalt environments provide a platform to better understand the catalytic activity of cobalt-based materials in the OER. Interestingly, among the four candidates, we find that Na 2 CoP 2 O 7 with T d geometry has excellent catalytic activity and high stability comparable to those of the well-known amorphous Co-Pi. Cyclic voltammetry (CV), high-resolution transmission electron microscopy (HR-TEM), X-ray photoelectron spectroscopy (XPS) and in-situ X-ray absorption near edge spectroscopy (XANES), scanning transmission electron microscopy energy-dispersive X-ray spectroscopy (STEM-EDX) and electron paramagnetic resonance (EPR) confirms the catalytic and structural stability of Na 2 CoP 2 O 7 . Theoretical calculations reveal that a unique OER pathway is present for Na 2 CoP 2 O 7 , which uses four coordinated cobalt atoms with low-energy barriers for the water-splitting reaction. Cobalt phosphates as a new group of OER catalysts The Na 2 CoP 2 O 7 , Li 2 CoP 2 O 7 , NaCoPO 4 and LiCoPO 4 compounds were synthesized using conventional solid-state methods, as described previously [41] , [42] , [43] , [44] , [45] , and the X-ray diffraction (XRD) patterns of the synthesized compounds well matched those of previous reports without impurites [41] , [42] , [43] , [44] , [45] ( Supplementary Fig. 1 ). The local crystal structure and overall networks of the polyhedrons in these four materials are schematically shown in Fig. 1 based on Rietveld analysis of each material along with the lattice parameters ( Supplementary Fig. 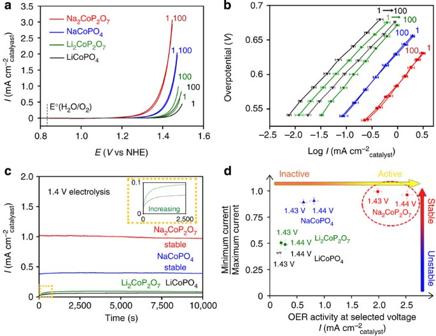Figure 2: Oxygen evolution performances of cobalt phosphate catalysts. (a) CV curves and (b) Tafel plots of Na2CoP2O7, Li2CoP2O7, NaCoPO4and LiCoPO4for the 1st and 100th cycle from 0.7 to 1.5 V versus NHE. The thermodynamic potential for water oxidation is marked at 0.816 V versus NHE (pH 7.0). (c) Bulk electrolysis was performed under a constant potential of 1.4 V versus NHE. The inset displays the enlarged bulk electrolysis profiles of Li2CoP2O7and LiCoPO4. (d) The electrochemical performances of Na2CoP2O7, Li2CoP2O7, NaCoPO4and LiCoPO4with respect to their catalytic activities and stabilities. OER current of 100th cycle at the selected voltage and the ratio of the minimum current to maximum current at the selected voltage during 100 cycles are depicted along thexaxis andyaxis, respectively. Error bars represent s.d. (n=5). 1 and Supplementary Table 2 ). Figure 1: Crystal structure and cobalt crystal field of cobalt phosphate catalysts. Crystal structures of ( a ) Na 2 CoP 2 O 7 , ( b ) Li 2 CoP 2 O 7 , ( c ) NaCoPO 4 and ( d ) LiCoPO 4 . The inset shows the local environment around the cobalt subunit (blue) and the spin state of the cobalt atom. The phosphate units, Na atoms and Li atoms are depicted in grey, yellow and green, respectively. Full size image The phosphate and pyrophosphate groups in these four materials induced various cobalt coordination and local polyhedron networks. Specifically, Na 2 CoP 2 O 7 and Li 2 CoP 2 O 7 have T d and mixed O h /TBP cobalt geometries, respectively, whereas the cobalt in NaCoPO 4 and LiCoPO 4 was only in the O h . T d polyhedron with higher point symmetry in Na 2 CoP 2 O 7 is not usual considering the fact that Co(II) is typically stabilized in O h environments [27] , [28] , [29] . Moreover, the T d polyhedrons are isolated by pyrophosphate groups, and with respect to the long-range ordering of the polyhedron the T d polyhedra in Na 2 CoP 2 O 7 form a two-dimensional layer via pyrophosphate groups, which is alternately stacked with sodium layers. Similarly, NaCoPO 4 exhibited a two-dimensional nature; however, each edge-sharing O h layer was cross-linked by a phosphate ligand. LiCoPO 4 exhibited similar structures as NaCoPO 4 in that two-dimensional chains of corner-sharing CoO 6 were linked by a phosphate ligand. However, in Li 2 CoP 2 O 7 , Co 2 O 9 subunits were interconnected through P 2 O 7 groups to build a 3D framework structure. These various structural features differ from the well-studied edge-shared O h CoO 6 observed in most cobalt-based catalysts [8] , [26] , [27] , [28] , [32] , [33] , [34] . OER catalytic behaviour of the cobalt phosphate catalysts The water oxidation catalytic properties of Na 2 CoP 2 O 7 , Li 2 CoP 2 O 7 , NaCoPO 4 and LiCoPO 4 were evaluated by CV in 0.5 M sodium phosphate buffer at pH 7.0 using a previously reported method [21] , [23] . One hundred cycles of potential sweep from 0.7 to 1.5 V versus normal hydrogen electrode (NHE) were performed for each substrate ( Supplementary Fig. 2 ). The 1st and 100th CV curves of Na 2 CoP 2 O 7 , Li 2 CoP 2 O 7 , NaCoPO 4 and LiCoPO 4 are shown in Fig. 2a . We observed that the catalytic activities increased in the series of LiCoPO 4 <Li 2 CoP 2 O 7 <NaCoPO 4 <Na 2 CoP 2 O 7 . Na 2 CoP 2 O 7 exhibited a current density of 2.62 mA cm −2 at 1.44 V versus NHE, which is significantly higher than those of NaCoPO 4 (0.90 mA cm −2 ), Li 2 CoP 2 O 7 (0.14 mA cm −2 ) and LiCoPO 4 (0.08 mA cm −2 ) under identical conditions. The superior catalytic activity of Na 2 CoP 2 O 7 compared with the other compounds was maintained even after 100 cycles. The activities of both Na 2 CoP 2 O 7 and NaCoPO 4 remained nearly unchanged during 100 cycles, whereas those of Li 2 CoP 2 O 7 and LiCoPO 4 slightly increased. The current densities of Li 2 CoP 2 O 7 and LiCoPO 4 changed from 0.14 to 0.29 mA cm −2 and from 0.08 to 0.19 mA cm −2 during 100 cycles at 1.44 V versus NHE, respectively. A similar current increase was previously observed in LiCoPO 4 (ref. 27 ), which was explained by the phase transformation on the catalyst surface, as will be discussed in detail in the later section. Figure 2: Oxygen evolution performances of cobalt phosphate catalysts. ( a ) CV curves and ( b ) Tafel plots of Na 2 CoP 2 O 7 , Li 2 CoP 2 O 7 , NaCoPO 4 and LiCoPO 4 for the 1st and 100th cycle from 0.7 to 1.5 V versus NHE. The thermodynamic potential for water oxidation is marked at 0.816 V versus NHE (pH 7.0). ( c ) Bulk electrolysis was performed under a constant potential of 1.4 V versus NHE. The inset displays the enlarged bulk electrolysis profiles of Li 2 CoP 2 O 7 and LiCoPO 4 . ( d ) The electrochemical performances of Na 2 CoP 2 O 7 , Li 2 CoP 2 O 7 , NaCoPO 4 and LiCoPO 4 with respect to their catalytic activities and stabilities. OER current of 100th cycle at the selected voltage and the ratio of the minimum current to maximum current at the selected voltage during 100 cycles are depicted along the x axis and y axis, respectively. Error bars represent s.d. ( n =5). Full size image The observed catalytic trend was also confirmed for the Tafel and potentiostatic electrolysis ( Fig. 2b,c and Supplementary Fig. 3 ). Figure 2b shows that the exchange current increases in the series of LiCoPO 4 <Li 2 CoP 2 O 7 <NaCoPO 4 <Na 2 CoP 2 O 7 , where the exchange currents are high for NaCoPO 4 and Na 2 CoP 2 O 7 even after 100 cycles of CV scans. The Tafel slopes of Na 2 CoP 2 O 7 , NaCoPO 4 , Li 2 CoP 2 O 7 and LiCoPO 4 at the 100th cycle were calculated as 82, 85, 84 and 82 mV dec −1 , respectively. Figure 2c indicates that the current densities of Na 2 CoP 2 O 7 and NaCoPO 4 in the potentiostatic electrolysis were stably maintained at a high value under constant potential 1.4 V versus NHE; in contrast, those of Li 2 CoP 2 O 7 and LiCoPO 4 were almost an order lower even though they slightly increased at the beginning of the electrolysis. It was found that the catalytic performance of Na 2 CoP 2 O 7 was almost comparable to that of the electro-deposited Co-Pi in Supplementary Fig. 4 . Despite the lower non-catalytic current, which is related to the number of redox-active cobalt ions or electrochemically active surface area [28] , [46] , the OER current of Na 2 CoP 2 O 7 was higher than that of the electro-deposited Co-Pi at 1.4 V versus NHE ( Supplementary Fig. 4 ). Comparison with β-CoOOH whose local structure is similar to that of Co-Pi exhibited similar trends (see details in the later part of the manuscript). However, it should be noted that, as Na 2 CoP 2 O 7 was synthesized using a conventional solid-state reaction and not by electrodeposition, a further study for comparing the catalytic abilities of the two samples using a similar preparation method is needed. In Fig. 2d , we summarized the electrochemical performance of four materials with respect to their catalytic activities and stabilities, that is, OER current after 100 cycles and the ratio of minimum to maximum current during the 100 cycles. A higher OER current along the x axis indicates a more active nature of the catalyst. Likewise, a higher current ratio close to unity along the y axis indicates better stability. As shown in Fig. 2d , Na 2 CoP 2 O 7 exhibits the best catalytic activity and stability among the four materials. Moreover, further long-term stability tests for Na 2 CoP 2 O 7 revealed that the catalytic current can be stably maintained during 500 cycles of CV scans and 12 h of bulk electrolysis ( Supplementary Fig. 5 ). In the following, a more detailed investigation is focused primarily on Na 2 CoP 2 O 7 . For deeper investigation of the OER performance of Na 2 CoP 2 O 7 , CV curves of Na 2 CoP 2 O 7 were recorded under various pH conditions from pH 5 to pH 13. As shown in Fig. 3a , the onset potential for Na 2 CoP 2 O 7 shifted towards a more negative potential with an increase in pH. The catalytic current was stably maintained during the OER under basic condition, whereas degradation in the catalytic current was observed during the OER tests at pH 5 ( Supplementary Fig. 6 ). 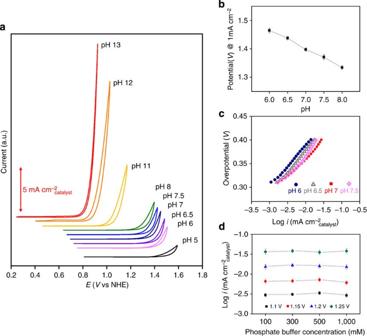Figure 3: OER catalytic performances of Na2CoP2O7at various pH and phosphate buffer concentrations. (a) CV curves for Na2CoP2O7from pH 5 to pH 13. (b) pH-dependent potential change at a constant current density of 1 mA cm−2. (c) Tafel plots of Na2CoP2O7from pH 6 to pH 7.5. (d) Phosphate buffer concentration dependency of the OER current at a constant applied potential (1.10, 1.15, 1.2 and 1.25 V versus NHE) at pH 7. Error bars represent s.d. (n=5). Figure 3: OER catalytic performances of Na 2 CoP 2 O 7 at various pH and phosphate buffer concentrations. ( a ) CV curves for Na 2 CoP 2 O 7 from pH 5 to pH 13. ( b ) pH-dependent potential change at a constant current density of 1 mA cm −2 . ( c ) Tafel plots of Na 2 CoP 2 O 7 from pH 6 to pH 7.5. ( d ) Phosphate buffer concentration dependency of the OER current at a constant applied potential (1.10, 1.15, 1.2 and 1.25 V versus NHE) at pH 7. Error bars represent s.d. ( n =5). Full size image The OER kinetics of Na 2 CoP 2 O 7 was examined by varying the pH and the phosphate concentration of the electrolytes ( Fig. 3a ). First, we investigated the pH-dependent potential change at a constant current density for understanding the dependence of the reaction rate on proton activity [47] , [48] , [49] . A plot between the pH and applied potential at constant current density of 1 mA cm −2 exhibited linearity from pH 6.0 to 8.0 and the slope was calculated as approximately −67 mV per pH ( Fig. 3b ). The Tafel slopes for pH 6, 6.5 and 7.5 were measured as ∼ 80 mV dec −1 , similar to the value at pH 7 ( Fig. 3c ). Then, the dependence of the reaction rate on the proton activity was derived by following equation [47] , [48] , [49] : Substituting and into the equation (1) leads to . This result indicated that the reaction rate follows an approximately inverse first-order dependence on the proton activity [47] , [48] , [49] . In addition, the dependence of the reaction rate on the phosphate-buffer strength was also examined by varying the buffer strength from 100 mM to 1 M. No change in the catalytic current depending on the buffer strength was found, indicating zero-order dependence on the phosphate-buffer strength ( Fig. 3d ) [47] , [48] . Although the measured Tafel slopes were somewhat far from 2.3 RT F −1 , typically 60 ∼ 80 mV dec −1 of Tafel slopes indicate that a one electron-transfer step is involved before rate determinant step (RDS) [48] , [49] . The exact reason for the higher Tafel values of our materials than 2.3 RT F −1 is unclear, but one possible explanation is that limitation in ion or electron transport might inflate the Tafel slope, as proposed in previous reports for LiCoPO 4 and thick Co-Pi films [27] . Although there is some deviation between the theoretical values and our experimental values, based on the Tafel and pH-dependent analysis, we can postulate that a one-proton/one-electron-involved equilibrium step may exist before the RDS in the OER mechanism of Na 2 CoP 2 O 7 (refs 47 , 48 , 49 ). Considering the calculated RDS of Na 2 CoP 2 O 7 was Co(IV)=O formation, as described in a later section, we could expect that equilibrium between Co(II) and Co(III) is the prior step before the RDS in the OER. The Faradaic efficiency of Na 2 CoP 2 O 7 during OER was quantified using oxygen sensor system. About 60 μmol of O 2 was produced during the electrolysis at 1.4 V versus NHE at a period of 5,000 s with a Faradaic efficiency of around ∼ 100%, indicating the measured current by CV is originated from the OER ( Fig. 4a ). With its proven ability for OER, facile mass production of Na 2 CoP 2 O 7 powder using conventional synthesis methods and electrode-fabrication techniques enable us to produce large-scale oxygen evolution systems. The catalytic currents can be increased by integrating stacks of cells or by enlarging the size of the conducting substrate, and 180 mA of OER current can easily be acquired by stacking two cells with a geometric area of 64 cm −2 ( Supplementary Fig. 7 ). 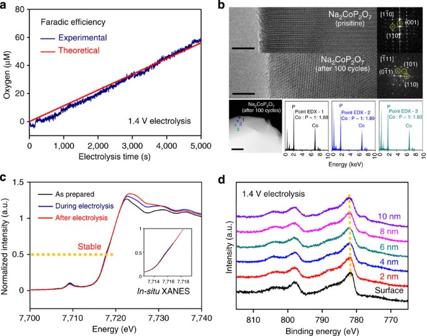Figure 4: Faradaic efficiency and structural stability of Na2CoP2O7during OER. (a) Faradic efficiency of Na2CoP2O7measured by an oxygen sensor system. Bulk electrolysis was performed in a gas-tight electrochemical cell with the O2sensor placed in the headspace. After initiating electrolysis at 1.4 V versus NHE, the percentage of O2measured in the sensor on the FOXY probe was converted into the partial pressure of O2in the headspace. The amount of evolved O2molecules detected during bulk electrolysis and the theoretical amount of evolved O2assuming a Faradaic efficiency of 100% are depicted by the blue line and red line, respectively. (b) HR-TEM images and FFTs at the surface region of Na2CoP2O7before and after 100 continuous potential cycles from 0.7 to 1.5 V versus NHE (scale bar, 5 nm). STEM image of Na2CoP2O7after potential cycles and point EDX spectrum from the surfaces to the inside region, showing similar Co/P ratios (scale bar, 20 nm). (c)In-situXANES spectra corresponding to the Co K-edge of Na2CoP2O7before, during and after bulk electrolysis at an applied potential of 1.5 V versus NHE for 2 h. The inset displays the enlarged XANES edge region. (d) XPS spectra of the Co 2pregion of the surface of the bulk-electrolysed sample at an applied potential of 1.4 V versus NHE for 1 h. Figure 4: Faradaic efficiency and structural stability of Na 2 CoP 2 O 7 during OER. ( a ) Faradic efficiency of Na 2 CoP 2 O 7 measured by an oxygen sensor system. Bulk electrolysis was performed in a gas-tight electrochemical cell with the O 2 sensor placed in the headspace. After initiating electrolysis at 1.4 V versus NHE, the percentage of O 2 measured in the sensor on the FOXY probe was converted into the partial pressure of O 2 in the headspace. The amount of evolved O 2 molecules detected during bulk electrolysis and the theoretical amount of evolved O 2 assuming a Faradaic efficiency of 100% are depicted by the blue line and red line, respectively. ( b ) HR-TEM images and FFTs at the surface region of Na 2 CoP 2 O 7 before and after 100 continuous potential cycles from 0.7 to 1.5 V versus NHE (scale bar, 5 nm). STEM image of Na 2 CoP 2 O 7 after potential cycles and point EDX spectrum from the surfaces to the inside region, showing similar Co/P ratios (scale bar, 20 nm). ( c ) In-situ XANES spectra corresponding to the Co K-edge of Na 2 CoP 2 O 7 before, during and after bulk electrolysis at an applied potential of 1.5 V versus NHE for 2 h. The inset displays the enlarged XANES edge region. ( d ) XPS spectra of the Co 2 p region of the surface of the bulk-electrolysed sample at an applied potential of 1.4 V versus NHE for 1 h. Full size image Structural and chemical stability of Na 2 CoP 2 O 7 during OER To understand the relative stability of Na 2 CoP 2 O 7 and NaCoPO 4 compared with the other two compounds during OER cycles, XRD analysis was performed. The XRD patterns in Supplementary Fig. 8 reveal no appreciable peak changes after the electrolysis. For detecting the possible structural changes at the surface, we performed surface-sensitive HR-TEM and XPS analysis on the electrolysed samples. The HR-TEM image and Fast Fourier Transform of Na 2 CoP 2 O 7 reveal the high crystallinity at the surface after 100 cycles ( Fig. 4b ). In addition, the NaCoPO 4 exhibited high crystallinity, as shown in Supplementary Fig. 9 . Point EDX analysis for bulk-electrolysed Na 2 CoP 2 O 7 in Cs-corrected STEM mode showed no change in the Co/P ratio from the surface to the bulk region, further supporting their structural stabilities. In contrast, an amorphous phase was formed on the surfaces of Li 2 CoP 2 O 7 and LiCoPO 4 after 100 potential cycles, whereas high crystallinity was found in pristine samples ( Supplementary Fig. 10 ). This observation is in good agreement with a previous study on LiCoPO 4 , which gradually amorphized from the surface, resembling the local structure of Co-Pi (ref. 27 ). Moreover, the point EDX spectra for the bulk-electrolysed Li 2 CoP 2 O 7 and LiCoPO 4 showed that the Co/P ratio of the amorphized surface region is ∼ 2, which is well accordant to that of Co-Pi (refs 8 , 27 ). In contrast, the bulk crystalline regions of Li 2 CoP 2 O 7 and LiCoPO 4 have Co/P ratios of 0.5 and 1, respectively, which were matched to their bulk compositional ratios. In addition, the CV curves for Li 2 CoP 2 O 7 , LiCoPO 4 and Co-Pi showed similar redox features before the catalytic waves and onset-potential voltage ( Supplementary Fig. 11 ). From the amorphous character and electrochemically similar behaviours of Li 2 CoP 2 O 7 , LiCoPO 4 and Co-Pi, it can be deduced that the surface structure undergo phase transformation into Co-Pi or Co-Pi analogues. Previous reports showed similar phase transformation into Co-Pi-like structures in LiCoPO 4 and Ba x Sr 1– x Co 0.8 Fe 0.2 O 3– δ during OER tests [27] , [28] . The high crystallinity and stability both at the surface and in the bulk of Na 2 CoP 2 O 7 and NaCoPO 4 are quite inspiring considering that most cobalt-containing materials undergo a transformation into an amorphous Co-Pi-like phase from the surfaces [27] , [28] , [30] . In-situ XANES and XPS analysis of Na 2 CoP 2 O 7 were performed to probe any irreversible variation of the cobalt valence states during the OER using an in-situ electrochemical cell [20] , [50] . The Co K-edge spectra of Na 2 CoP 2 O 7 were measured from 2 to 3 h after initiation of electrolysis at 1.5 V versus NHE. The Co K-edge spectra remained nearly constant during and after bulk electrolysis at 1.5 V versus NHE ( Fig. 4c ), indicating that no major change in the cobalt oxidation state occurred. In contrast to Na 2 CoP 2 O 7 , the Co K-edge spectra of the electrolysed Li 2 CoP 2 O 7 and LiCoPO 4 shifted towards the higher-energy region compared with that of the as-prepared sample, implying that cobalt oxidation occurred during the OER ( Supplementary Fig. 12 ). Moreover, the Co 2p XPS peaks from the surface to a depth of 10 nm of the bulk-electrolysed Na 2 CoP 2 O 7 and NaCoPO 4 showed negligible variation ( Fig. 4d and Supplementary Fig. 13 ). In contrast, the XPS depth profiling from the surface to 12-nm depths of cycled Li 2 CoP 2 O 7 and LiCoPO 4 showed that the surface Co 2 p peaks shifted towards higher energy compared with those of the bulk, further supporting their structural change on electrolysis ( Supplementary Fig. 13 ). EPR analysis clearly showed the different structural stabilities of Na 2 CoP 2 O 7 , NaCoPO 4 , Li 2 CoP 2 O 7 and LiCoPO 4 during the OER tests by direct observations of Co(II) and Co(IV) species. The continuous-wave X-band EPR spectrum for Na 2 CoP 2 O 7 only exhibited a characteristic S =3/2, Co(II) signal at g eff ≈5 after bulk electrolysis at various potentials and times ( Fig. 5a ). Even 300 min of bulk electrolysis at 1.4 V versus NHE did not trigger a change in the Co EPR signal. Here, the signal at g =2 resulted from the carbon support ( Supplementary Fig. 14 ). Invariance of the EPR signals on electrolysis supported the high structural stability of Na 2 CoP 2 O 7 . 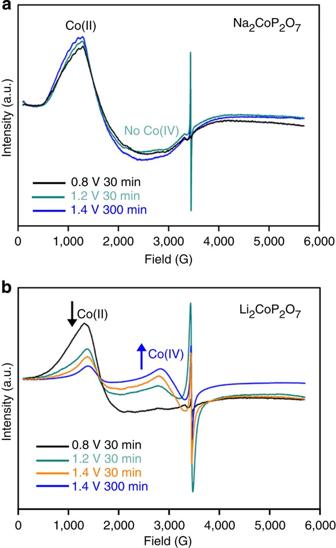Figure 5: Continuous wave X-band EPR spectra for Na2CoP2O7and Li2CoP2O7on bulk electrolysis. (a) EPR spectra for Na2CoP2O7at 0.8 V for 30 min (black), 1.2 V for 30 min (green) and 1.4 V for 300 min (blue). Only Co(II) signals atgeff≈5 appeared on bulk electrolysis. Here, the signal atg=2 is originated from carbon. (b) EPR spectra for Li2CoP2O7at 0.8 V for 30 min (black), 1.2 V for 30 min (green), 1.4 V for 30 min (orange) and 1.4 V for 300 min (blue). Contrary to Na2CoP2O7, a decrease in Co(II) signals with a concurrent increase in Co(IV) signals (geff≈2.3) was observed with the increase in applied voltage and time. Figure 5: Continuous wave X-band EPR spectra for Na 2 CoP 2 O 7 and Li 2 CoP 2 O 7 on bulk electrolysis. ( a ) EPR spectra for Na 2 CoP 2 O 7 at 0.8 V for 30 min (black), 1.2 V for 30 min (green) and 1.4 V for 300 min (blue). Only Co(II) signals at g eff ≈5 appeared on bulk electrolysis. Here, the signal at g =2 is originated from carbon. ( b ) EPR spectra for Li 2 CoP 2 O 7 at 0.8 V for 30 min (black), 1.2 V for 30 min (green), 1.4 V for 30 min (orange) and 1.4 V for 300 min (blue). Contrary to Na 2 CoP 2 O 7 , a decrease in Co(II) signals with a concurrent increase in Co(IV) signals ( g eff ≈2.3) was observed with the increase in applied voltage and time. Full size image In contrast, the distinct EPR signal around g eff ≈2.3, which can be assigned to the low spin Co(IV) with its total spin S =1/2, appeared on bulk electrolysis of Li 2 CoP 2 O 7 at an applied voltage of above 1.2 V versus NHE. With the decrease in the Co(II) signal, the Co(IV) signal increased when we raised the applied potential or electrolysis time, suggesting that significant oxidation of Co(II) into Co(IV) in Li 2 CoP 2 O 7 occurred during the OER ( Fig. 5b ). Similar EPR trends were observed in previous reports using Co-Pi and they found that its catalytic resting state comprises Co(IV) species [30] , [51] . The increase in the Co(IV) signal with the concurrent decrease in Co(II) presented another evidence for structural change of Li 2 CoP 2 O 7 into Co(IV)-containing Co-Pi-like structures during OER. Similar with the case of Na 2 CoP 2 O 7 and Li 2 CoP 2 O 7 , the EPR spectrum for bulk-electrolysed NaCoPO 4 only showed a Co(II) signal at g eff ≈5, whereas a distinct Co(IV) signal at g eff ≈2.3 was found in bulk-electrolysed LiCoPO 4 ( Supplementary Fig. 15 ). In our studies the Co(III) signal did not appear, because the low-spin Co(III) with its total spin S =0 is EPR silent and high-spin Co(III) are rare and only existed in weak-field ligands, as described previously [51] . Although it is uncertain whether a small portion of Co(II) in Na 2 CoP 2 O 7 or NaCoPO 4 transformed into Co(III) during the OER, based on negligible change in the Co(II) signal on bulk electrolysis and no appearance of a Co(IV) signal, we believe that their dominant Co species during OER may be Co(II) or Co(II)/Co(III) mixed states. In addition, these EPR results supported phase transformation of Li 2 CoP 2 O 7 and LiCoPO 4 during the OER into Co(IV)-containing Co-Pi-like structures. Calculated surface structures of Na 2 CoP 2 O 7 To understand the catalytic activity of Na 2 CoP 2 O 7 with respect to its local structure on an atomistic level, we performed a series of first-principles calculations. The possible surface structures of Na 2 CoP 2 O 7 were first calculated to estimate the equilibrium morphology at pH 7.0 ( Supplementary Table 3 ). Based on the relative surface energies, the equilibrium crystal shape of Na 2 CoP 2 O 7 was projected using Wulff constructions, which revealed that Na 2 CoP 2 O 7 is mainly composed of a (101) surface with slight (001) surface exposure ( Fig. 6a ). It is worth noting that in the main (101) surface of Na 2 CoP 2 O 7 , the pyrophosphate ligands rotated around the cobalt atoms and generated a new Co–O bond, as illustrated in Fig. 6b . As shown in Supplementary Fig. 16 , a general relaxation of surface atoms occurred and then new Co–O bonds were formed by rotation of the pyrophosphate ligands. After new Co–O bonds were formed, further relaxation occurred, creating the final surface structures of Na 2 CoP 2 O 7 (101) plane. It should be noted that the pyrophosphate-group rotation in surface spontaneously occurs following an energetically favourable pathway with the decrease of Gibbs free energy. The structural flexibility of the P 2 O 7 group could stabilize the under-coordinated transition metals on the surface [40] . As a result of the passivation by the pyrophosphate group, three-coordinated surface cobalt atoms initially formed after surface-cleaving step irreversibly transformed into a highly distorted tetrahedral geometry similar to the CoO 5 TBP structure with a deficiency of one oxygen. 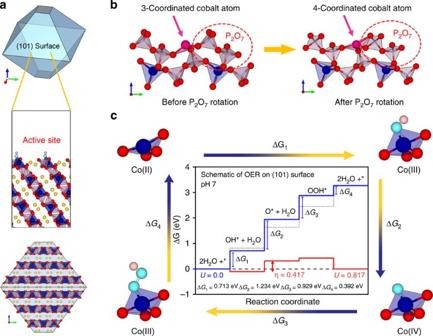Figure 6: Density functional theory calculation for OER mechanism of Na2CoP2O7. (a) Wulff structure of Na2CoP2O7, showing the equilibrium crystal shape based on the relative surface energies and the enlarged (101) surface with active sites. (b) Local environment around the active cobalt atom located on the (101) surface before and after P2O7rotation; the active cobalt atom is depicted in pink. (c) Schematic of the Gibbs free energy changes for the four elementary steps during the OER based on DFT calculations. The local structure and valence change of the cobalt atoms in the active sites are shown at the corners. The inset shows the free-energy landscape on the (101) surface of Na2CoP2O7compared with an ideal catalyst at pH 7.0. An ideal catalyst, Na2CoP2O7forU=0 and Na2CoP2O7forU=0.817 are depicted by the dashed line, blue line and red line, respectively. Figure 6: Density functional theory calculation for OER mechanism of Na 2 CoP 2 O 7 . ( a ) Wulff structure of Na 2 CoP 2 O 7 , showing the equilibrium crystal shape based on the relative surface energies and the enlarged (101) surface with active sites. ( b ) Local environment around the active cobalt atom located on the (101) surface before and after P 2 O 7 rotation; the active cobalt atom is depicted in pink. ( c ) Schematic of the Gibbs free energy changes for the four elementary steps during the OER based on DFT calculations. The local structure and valence change of the cobalt atoms in the active sites are shown at the corners. The inset shows the free-energy landscape on the (101) surface of Na 2 CoP 2 O 7 compared with an ideal catalyst at pH 7.0. An ideal catalyst, Na 2 CoP 2 O 7 for U =0 and Na 2 CoP 2 O 7 for U =0.817 are depicted by the dashed line, blue line and red line, respectively. Full size image OER catalytic mechanism of Na 2 CoP 2 O 7 Given the well-established surface structures, we attempted to estimate the overpotential by sequentially calculating the Gibbs free energies for the four elementary steps occurring on the surface during the OER based on acid–base mechanism [18] , [22] , [31] . These four steps are used for modelling the thermochemistry of the OER [18] , [22] , [31] and are described as follows: (*represents the active surface site where OH and O species can adsorb). During the process, water molecules first adsorb on the active site on the surface and dissociate into a proton and OH* (step 1), which again splits into a proton and O* (step 2). The oxygen atom recombines with a water molecule to form an OOH* bond (step 3) and finally evolves as O 2 gas (step 4). Our calculation model has limitations in neglecting the influence of the electric field on the double layer and the possible differences resulting from the types of proton donor (H 3 O + or H 2 O). According to previous reports [18] , [52] , [53] , with this assumption, the Gibbs free energy of each step during the OER can be calculated as identical, regardless of the pH value. In this regard, we simply calculated the Gibbs free energy of each step in Na 2 CoP 2 O 7 using the four-step model in acidic conditions. Moreover, it should be noted that an alternative OER mechanism exists, the so-called direct coupling mechanism [54] , [55] . Recently, Wang and Van Voorhis [54] revealed the new OER mechanism in cobalt oxide, demonstrating direct-coupling O–O bond formation can occur with a very low activation barrier, and steps other than O–O bond formation act as the RDS in cobalt oxides. In this stage, based on the relatively larger inter-cobalt distance in Na 2 CoP 2 O 7 (5.15 Å) compared with that in cobalt oxide ( ∼ 2.85 Å) revealed by in-situ XAS analysis [26] , we focused on the acid–base mechanism for exploring the OER pathway in Na 2 CoP 2 O 7 . During these four steps, the cobalt ion is sequentially oxidized from 2 to 3 (step 1) and 3 to 4 (step 2), and is reduced from 4 to 3 (step 3) and 3 to 2 (step 4), indicating the active participation of the cobalt redox reaction at every step of the OER. The detailed energy changes during the four elementary steps are shown for the two dominant surfaces, (101) and (001) surfaces, in Fig. 6c and Supplementary Fig. 17 , respectively. Here, the dotted line represents the calculated Gibbs free energies at ideal charge transfer steps and the blue line represents those of Na 2 CoP 2 O 7 when U =0, both at pH 7.0. The red line represents the net Gibbs free energy changes of Na 2 CoP 2 O 7 when U =0.817, which represents the additionally required energy for the reaction to proceed (equivalent to the overpotential) in each step during the OER. Probing the Gibbs free energies for these steps reveals that the (101) surface exhibits a significantly lower overpotential of 0.417 eV than that of the (001) surface of 1.117 eV ( Fig. 6c and Supplementary Fig. 17 ). It is noteworthy that the magnified CV curves in Supplementary Fig. 4 show that the current increased dramatically near the overpotential of 0.42 V, supporting the validity of our calculations, although experimental overpotential may slightly vary with the current density. The individual steps of the water oxidation are closely investigated in the following. As a first step, we monitored the Gibbs free energy change for OH* formation (step 1) on the (101) surface in our system. As the absorption of water molecules on the surface is the initial step of the OER, it is generally perceived that the absorption energy of water molecules highly affects the OER activity [52] , [53] , [54] , [55] , [56] , [57] , [58] , [59] , [60] . Norskov and colleagues [52] , [53] , [58] reported the importance of the adsorption energies of adsorbents, such as *OH and *OOH species, on the OER activities on metal-oxide surfaces and a universal scaling relation between *OH and *OOH adsorption energy was found. Recently, Liu et al . [59] and Kim et al . [60] showed that oxygen or cobalt vacancies with high binding energies with water molecules lead to a significant enhancement of OER catalytic capabilities. Interestingly, the Gibbs free energy for step 1 in our system only requires 0.713 eV, which is lower than the energy needed (0.817 eV) to initiate water oxidation ideally at pH 7.0, implying a facile water adsorption on surface cobalt atoms in the (101) plane. This facile adsorption originates from the unique structural characteristic of the reorganized surface cobalt atoms; pyrophosphate ligands induced highly distorted T d coordination, which has an open site, where oxygen adsorbants can easily bind. Indeed, previous reports showed that similar distorted metal geometries with open coordination sites have an advantage in the uptake of oxygen adsorbants [59] , [60] , [61] , [62] . This finding strongly suggests that the distorted local cobalt geometry induced by the reorganization of pyrophosphate ligands contributed to a favourable water adsorption and further water oxidation catalysis. Compared with facile OH* formation, O* formation (step 2) requires the highest barrier (0.417 eV) among the four steps, indicating that this step is the rate-limiting process of the water oxidation catalysis of Na 2 CoP 2 O 7 . This theoretical value is comparable in magnitude to that of the active cobalt-oxide β-CoOOH (0.48 eV), which was selected as a representative for amorphous Co-Pi (ref. 31 ). Considering that RDS in conventional cobalt oxides including β-CoOOH is generally known as OOH* formation [30] , [31] , the limiting step of O* formation in Na 2 CoP 2 O 7 is worthwhile to be noticed. However, it should be noted that steps other than O–O bond formation can be the RDS by direct O–O coupling [54] . We speculate that the highest barrier residing in step 2 of Na 2 CoP 2 O 7 is related to the inherent nature of the high cobalt oxidation potential in the phosphate framework [42] , [43] , [45] . Much higher redox potentials for cobalt (Co(II)/Co(III) or Co(III)/Co(IV)) are generally observed in polyanion frameworks such as phosphates and pyrophosphates compared with oxides because of the inductive effect [42] , [43] , [45] . As step 2 requires the oxidation of the Co(III) to Co(IV) in pyrophosphates, a substantially higher energy will be required to oxidize the Co(III) ion than in oxides [42] , [43] , [45] . It is noteworthy that the redox potentials of cobalt ions in oxides typically shift up by ∼ 1 V in phosphates [42] , [45] . The higher energy for oxidizing Co(III) in Na 2 CoP 2 O 7 may make O* formation the RDS. Another interesting characteristic of Na 2 CoP 2 O 7 was found in the adaptable local cobalt structure during the OER (corners of Fig. 6c ). Although the OER proceeds in five- and six-coordinated polyhedron in conventional cobalt oxides [26] , [30] , [31] , Na 2 CoP 2 O 7 used four- and five-coordination geometries accompanying the change of cobalt valence. Specifically, with the valence change from 2 to 3 in step 1, the oxygen coordination number of cobalt increased from 4 to 5 by adsorbing the OH species. Then, further oxidation to Co(IV) occurs by detaching the proton from the adsorbed OH and the remaining oxygen bound to Co(IV) recombines with a water molecule to make OOH, reducing the cobalt to III. During these two redox steps (step 2 and 3), the five-coordination geometry was retained without a significant change in the atom positions. As under-coordinated transition metals are generally unstable and are prone to induce surface reconstruction [63] , [64] , the stable performance of the four/five coordination of cobalt is remarkable. This performance was possible mainly because of the rotation of the flexible pyrophosphate group, which readily forms additional Co–O bonds at the surface, indicating the important interplay between the cobalt ion and phosphate polyanion. We performed additional computations to explore the theoretical OER mechanism for NaCoPO 4 and β-CoOOH ( Supplementary Fig. 18 ). β-CoOOH was introduced for representing Co-Pi-like structures at the surface of Li 2 CoP 2 O 7 and LiCoPO 4 during the OER. The four OER steps of the dominant NaCoPO 4 surface, the (010) plane, showed that theoretical overpotential of NaCoPO 4 was 0.60 V with RDS of O* formation. In case of β-CoOOH, the plane was selected as the most catalytically active surface, on the basis of a previous study based on the acid–base mechanism. The theoretical overpotential of β-CoOOH was calculated as 0.44 V with RDS of *OOH formation, which was in line with a previous report [31] . Finally, we compared the similar and different characteristics of Na 2 CoP 2 O 7 and Co-Pi (β-CoOOH) in Table 1 . Whereas these two types of catalyst exhibited similar electrochemical performances, their underlying catalytic mechanisms showed strikingly different properties. In terms of structure, Na 2 CoP 2 O 7 has four/five-coordination geometry inside the crystalline structure during OER, whereas Co-Pi has O h -based five/six coordination in an amorphous structure [8] , [30] , [31] . The dominant Co species of Na 2 CoP 2 O 7 during OER is Co(II) or Co(II)/Co(III), whereas that of Co-Pi is known as Co(III)/Co(IV) [26] , [30] . Finally, the theoretically calculated RDE of Na 2 CoP 2 O 7 is *O formation, whereas that of Co-Pi is *OOH formation (acid–base mechanism) [30] , [31] . Based on these comprehensive comparisons, we think that Na 2 CoP 2 O 7 can be a good model system to explore new OER chemistry beyond conventional O h -based cobalt-oxide materials. Table 1 Comparison between Na 2 CoP 2 O 7 and CoO x . Full size table In summary, we explored the abilities of four phosphate/pyrophosphate-based, well-known cobalt redox-active materials as water oxidation catalysts and found a highly active and stable material, Na 2 CoP 2 O 7 . Whereas previously reported cobalt-containing materials underwent significant phase transformation during the OER, Na 2 CoP 2 O 7 exhibited excellent catalytic activity and phase stability. Moreover, mechanistic studies for the OER of Na 2 CoP 2 O 7 were performed by varying the pH and phosphate buffer strength of the electrolyte. Density functional theory calculations revealed that Na 2 CoP 2 O 7 have lower theoretical overpotential ( ∼ 0.42 eV) compared with the most active cobalt-oxide phase, CoOOH ( ∼ 0.48 eV), theoretically verifying its high catalytic activity. In addition, we found the possible OER pathway in Na 2 CoP 2 O 7 that used four- and five-coordinated cobalt atoms stabilized by actively rotating pyrophosphate groups. Through the experimental and theoretical comparison, we found that the underlying catalytic mechanism of Na 2 CoP 2 O 7 was notably different to that of the conventional cobalt oxides, in terms of RDS, local cobalt structure and cobalt valence state during the OER. We believe that using polyanion-based cobalt compounds can be an interesting new direction for the development of new efficient and stable catalysts, and the discovery of new catalytic pathways in various transition metal geometries. We expect that this result can broaden the current oxide-based picture of the water oxidation complex and give hints at a possible effect of the polyanion on OER catalytic abilities. Material synthesis Na 2 CoP 2 O 7 and NaCoPO 4 powders were synthesized using the conventional solid-state method. Stoichiometric amounts of Na 2 CO 3 (ACS reagent, ⩾ 99%, Aldrich), CoC 2 O 4 ( ⩾ 99%, Kojundo) and (NH 4 ) 2 HPO 4 (ACS reagent 98%, Aldrich) were wet-ball milled in acetone media and heated at 300 °C under Ar media for 6 h. After grinding, the pelletized samples were calcined at 600 °C and 750 °C under Ar media for 6 h for Na 2 CoP 2 O 7 and NaCoPO 4 , respectively. Li 2 CoP 2 O 7 and LiCoPO 4 powders were synthesized using the stoichiometric amounts of Li 2 CO 3 (ACS reagent, ⩾ 99%, Aldrich), CoC 2 O 4 ( ⩾ 99%, Kojundo) and (NH 4 ) 2 HPO 4 (ACS reagent 98%, Aldrich). The precursors were mixed by ball milling, heated at 300 °C under Ar media for 6 h, pelletized and calcined at 600 °C for Li 2 CoP 2 O 7 and 800 °C for LiCoPO 4 under Ar media for 6 h. Amorphous Co-Pi was synthesized according to the previous report [8] . Material characterization Powder XRD patterns were measured using a Bruker D-8 Advance X-ray diffractometer using Cu Kα radiation ( λ =1.54056 Å) from 10° to 70° with a step size of 0.01°. Structural analysis of materials was performed by Rietveld refinement method using FullProf software. TEM images were obtained using a field-emission TEM (Philips Tecnai F20) operating at 200 kV. HR-TEM images and FFTs of the materials were used to analyse surface morphology. Point EDX analysis was performed under the Cs-corrected STEM mode and the spectra from three different regions were acquired with a Quanta 3D FEG (FEI, The Netherlands). The XAS experiments were performed at beamline 8C at the Pohang Accelerator Laboratory, Republic of Korea. The oxidation state corresponding to the Co K-edge in each sample was investigated using XANES analysis. In-situ XANES spectra were collected in fluorescence mode with an electron energy of 2.5 GeV and stored in the current of 250 mA top-up mode. XPS spectra were performed to examine the oxidation state of the Co 2 p peaks from surface to depth of 10 nm of the catalyst after bulk electrolysis. XPS analysis was performed five times at an increment of 2 nm etching from the surface. The data were attained with passing energy 23.5 eV with a step size of 0.05 eV by electron spectroscopy (Sigma Probe, Thermo VG Scientific, UK). Brunauer–Emmett–Teller analysis was performed to analyse the surface area of the catalyst. The sample was loaded in the Brunauer–Emmett–Teller analyser (Tristar II 3020 Micromeritics, USA) under an N 2 adsorption environment. Electrochemistry The electrochemical measurements were performed in a three-electrode system using a potentiostat (CHI 760C, CH Instruments, Inc.). Pt foil (2 cm × 2 cm × 0.1 mm, 99.997% purity, Alfa Aesar) was used as the counter electrode and Ag/AgCl electrode (BASi, 3 M NaCl) was used as a reference electrode. The working electrode was prepared by a previously reported spin-coating method [21] , [23] . The catalyst with neutralized Nafion solution was dispersed in purified deionized water using sonication and was spin-coated onto an fluorine-doped tin oxide substrate. After the electrode was dried at 80 °C for 5 min, the loaded catalyst weight was carefully measured using a micro weighing electronic scale (Sartorius Micro Balance). A pH 7.0 sodium phosphate buffer with buffer strength 0.5 M was used as the electrolyte, and the electrolyte was degassed with high-purity N 2 before every electrochemical measurement. The OER curves were corrected using the averaged value of the forward and reverse CV currents for polarization compensation and further iR-compensation using V = V applied −iR was performed. After polarization and iR compensation, each OER value was normalized to the total surface area of the catalysts on the substrate. The electrochemical potentials were converted to the NHE scale by following equation: E (NHE)= E (Ag/AgCl)+0.197 V. To prepare electrolytes with different pH values from 5.0 to 8.8, 0.5 M phosphate buffer was used with varying ratios of NaH 2 PO 4 and Na 2 HPO 4 . Over pH 9, the pH was adjusted by addition of NaOH into the phosphate buffer (pH 8.8) in the customary manner. To determine the effect of the phosphate buffer concentration on the activity, different phosphate buffer concentrations from 0.1 to 1 M were prepared and different amounts of NaClO 4 were added to maintain the same solution conductivity regardless of the phosphate buffer concentrations. EPR measurement X-band continuous-wave EPR spectra were obtained using a Bruker EMX/Plus spectrometer equipped with a dual-mode cavity (ER 4116DM). A liquid He quartz cryostat (Oxford Instruments ESR 900) combined with gas flow controller (Oxford Instruments ITC 503) was introduced to control the low temperatures ( ∼ 5.7 K). For EPR measurement, 15 mg of Na 2 CoP 2 O 7 , NaCoPO 4 , Li 2 CoP 2 O 7 and LiCoPO 4 catalyst electrodes were prepared as carbon-paste type. After bulk electrolysis at the specific voltages and times, the electrodes were removed from electrolyte, followed by quick drying using an Ar (99.999 %) gun. Then, the solid-state catalysts were carefully collected by a razor blade and were transferred to an EPR tube under Ar (99.999 %) atmosphere. The EPR tube was immediately frozen and stored at 77 K using liquid nitrogen before EPR measurement. The elapsed time from the end of electrolysis to freezing of the EPR tube was ∼ 5 min. The following parameters were used: microwave frequency=9.64 GHz, modulation amplitude=10 G, modulation frequency=100 kHz, microwave power=0.94 mW and temperature=5.7 K. Ten scans were added for obtaining each spectrum. First-principles calculations All the free energies in this work were calculated using the generalized gradient approximation (GGA) and the Perdew–Burke–Ernzerhof functional for the exchange correlation to the density functional theory [65] . The projected augmented wave method was used, as implemented in the Vienna ab initio simulation package [66] . The Hubbard U parameter (GGA+ U ) with U =3.5 eV was used to accurately calculate the electron correlation within the d states in a cobalt ion [67] , [68] , [69] , [70] . A 3D slab model with periodic boundary conditions was used with an energy cutoff of 500 eV and an appropriate γ -point, only k -points mesh, was selected to ensure that the total energies converged within 5 meV per formula unit of Na 2 CoP 2 O 7 . Wulff construction and surface properties To calculate the surface energies and Wulff shape of Na 2 CoP 2 O 7 , the initial unrelaxed surface structures were carved out from the fully relaxed bulk structure of Na 2 CoP 2 O 7 with P42mnm symmetry, which is a less distorted structure with higher symmetry than the experimental P21cn structure. The selection of surfaces to investigate was limited to low-index surfaces and guided by favouring surfaces with preservation of the PO 4 tetrahedron, which led to the following set of surfaces: (100), (001), (110), (210), (101), (111) and . All the surface structures were calculated within the GGA+U scheme as defined above, using a supercell with atomic layers over 15 Å and vacuum slabs over 20 Å along the z direction using a convergence test to obtain the adsorption energies and to recover the bulk magnetic ordering of the centre layers (convergence within 1 meV Å −2 for the surface energies). The surface energies were calculated from equation (6) on either stoichiometric or non-stoichiometric slabs for which the top- and bottom-most cobalt pyrophosphate layers were relaxed below the force threshold of 0.05 eV Å −1 . with surface area 2A, free energy G slab , chemical potentials μ i , the number of excess adsorbed species over bulk N i − x i N Co (where x i is the number of atoms per bulk formula). The chemical potentials μ i of the adsorbents were taken relative to the free energy of liquid water and hydrogen gas, written explicitly as functions of pH and applied potential U: where U is the potential measured against NHE at standard conditions and Δ G H + (pH) is − k B T log(pH). Gibbs free energy changes in water oxidation steps We defined the OER steps similar to equations (2, 3, 4, 5) in the manuscript. The Gibbs free energy changes for the water oxidation steps (equations (2, 3, 4, 5) in the manuscript) were calculated using the following equations: where the density functional theory energies, zero point energy and entropy correction values are listed in the Supplementary Table 4 . How to cite this article: Kim, H. et al . Coordination tuning of cobalt phosphates towards efficient water oxidation catalyst. Nat. Commun. 6:8253 doi: 10.1038/ncomms9253 (2015).